Optical signatures of silicon-vacancy spins in diamond Colour centres in diamond have emerged as versatile tools for solid-state quantum technologies ranging from quantum information to metrology, where the nitrogen-vacancy centre is the most studied to date. Recently, this toolbox has expanded to include novel colour centres to realize more efficient spin-photon quantum interfaces. Of these, the silicon-vacancy centre stands out with highly desirable photonic properties. The challenge for utilizing this centre is to realize the hitherto elusive optical access to its electronic spin. Here we report spin-tagged resonance fluorescence from the negatively charged silicon-vacancy centre. Our measurements reveal a spin-state purity approaching unity in the excited state, highlighting the potential of the centre as an efficient spin-photon quantum interface. Diamond is a promising spin-free material for a range of novel technologies that make use of its optically accessible lattice impurities (colour centres). The most eminent colour centre in diamond to date, the negatively charged nitrogen-vacancy (NV) centre, has attracted great interest in recent years for quantum information processing [1] , [2] , [3] , electromagnetic field sensing [4] , [5] , [6] , [7] and biomarking [8] , [9] . The NV centre owes its success to the optically accessible spin triplet in the ground state with room temperature electron-spin coherence times of up to 2 ms in ultrapure bulk diamond [10] . This allows for initialization [11] , coherent control [12] , [13] , [14] , [15] and projective read-out [11] to be performed with high fidelity. However, for photon-based quantum communication architectures, the challenge for the NV centre and most other diamond colour centres is to overcome the fundamental limitation of only weak emission into the zero-phonon line (ZPL), for example, by incorporating them in nanophotonic cavities [16] . An alternative approach is to identify other centres with superior photonic (but comparable spin) properties to NV. Recent studies of such centres include chromium- [17] , [18] , xenon- [19] nickel- [20] and possibly oxygen-related centres [21] , as well as the negatively charged silicon-vacancy (SiV) centre [22] , [23] , [24] . The latter has the advantage of being the brightest reported colour centre in diamond [24] . Its emission is concentrated to about 80% into its ZPL even at room temperature [23] , thus making it a promising single-photon source. One major challenge is to achieve direct (optical) access to the electronic spin degree of freedom similar to that of NVs. Previous electron-spin resonance measurements on ensembles of neutrally charged SiV centres have identified an S =1 ground state [25] , [26] , [27] , suggesting strongly that the negatively charged centres should be associated with an S =1/2 ground state. However, optical access to this electronic spin has remained elusive for both charge states. Here, we report the direct accessing and spin-selective population of the negatively charged SiV centre excited states, achieved via resonant excitation and fluorescence under a magnetic field. In low-strain bulk diamond spin-selective excitation under finite magnetic field reveals a spin purity approaching unity in the excited state. We also investigate the effect of strain on the centres in nanodiamonds and discuss how spin selectivity in the excited state remains accessible in this regime. Characterization of the SiV − centre in a magnetic field The SiV centre in diamond consists of a silicon atom and a vacancy in a split-vacancy configuration [28] , [29] , [30] , replacing two neighbouring carbon atoms in a diamond matrix along the 111 axes (see Fig. 1a , inset). The substitutional silicon atom relaxes to the middle of the two lattice sites creating an inversion symmetric complex [29] , [31] . A total of 10 electrons are associated with this centre, as can be counted from the SiV structure in Fig. 1a , inset. One extra electron is captured to form the negatively charged complex (SiV − ). With 11 electrons in total, a single electron remains unpaired resulting in an effective spin-1/2 for the negatively charged state of the centre. 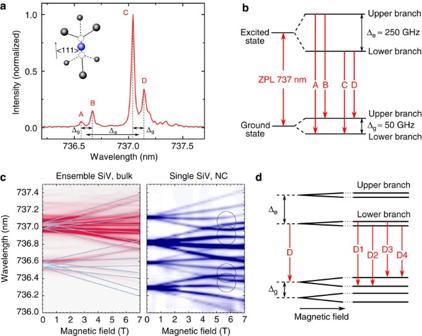Figure 1: Introduction to the SiV−centre. (a) Fluorescence spectrum at 4 K for an SiV−ensemble in [001]-oriented bulk diamond obtained by non-resonant excitation at 700 nm. The dominant transitions due to the28Si isotope, forming two doublets, are labelled from A to D, and the weaker, red-shifted transitions originate from29Si and30Si. The atomic structure of the SiV−centre is shown in the inset, with the silicon atom (blue) in split-vacancy configuration between the unoccupied lattice sites (dashed circles) and the nearest neighbour carbon atoms (grey). (b) Energy level scheme of the SiV−centre. The split ground and excited states give rise to four optical transitions, labelled from A to D according to the transitions ina. (c) Fluorescence spectra at 4 K as a function of magnetic field along [001] for an ensemble of SiV−centres in bulk diamond (red colour plot, light blue lines are a guide to the eye) and for a single SiV−in a diamond nanocrystal (blue colour plot), where the strain induces a larger splitting of the doublets at zero field, resulting in a clearer splitting into a quadruplet for each transition. Avoided crossings in the spectrum, marked by black dashed circles, originate from spin-orbit coupling31. (d) Magnetic field splitting of each spin-1/2 energy level. The optical transitions split into four as shown for transition D due to the different g-factors in the ground and excited states. Figure 1: Introduction to the SiV − centre. ( a ) Fluorescence spectrum at 4 K for an SiV − ensemble in [001]-oriented bulk diamond obtained by non-resonant excitation at 700 nm. The dominant transitions due to the 28 Si isotope, forming two doublets, are labelled from A to D, and the weaker, red-shifted transitions originate from 29 Si and 30 Si. The atomic structure of the SiV − centre is shown in the inset, with the silicon atom (blue) in split-vacancy configuration between the unoccupied lattice sites (dashed circles) and the nearest neighbour carbon atoms (grey). ( b ) Energy level scheme of the SiV − centre. The split ground and excited states give rise to four optical transitions, labelled from A to D according to the transitions in a . ( c ) Fluorescence spectra at 4 K as a function of magnetic field along [001] for an ensemble of SiV − centres in bulk diamond (red colour plot, light blue lines are a guide to the eye) and for a single SiV − in a diamond nanocrystal (blue colour plot), where the strain induces a larger splitting of the doublets at zero field, resulting in a clearer splitting into a quadruplet for each transition. Avoided crossings in the spectrum, marked by black dashed circles, originate from spin-orbit coupling [31] . ( d ) Magnetic field splitting of each spin-1/2 energy level. The optical transitions split into four as shown for transition D due to the different g-factors in the ground and excited states. Full size image We study two types of samples containing SiV − centres: a diamond film grown homoepitaxially via chemical vapour deposition (CVD) on a high pressure high temperature bulk diamond [32] and CVD-grown diamond nanocrystals on an Ir substrate [23] . The former offers a relatively homogenous low-strain environment preserving the intrinsic symmetry of the centre. On the other hand, the latter, from which the SiV − fluorescence can be extracted with high efficiency [24] , provides a strained environment modifying the emission properties from centre to centre [24] , [32] . At cryogenic temperatures, the photoluminescence spectrum of the ZPL reveals a characteristic fine structure composed of four transitions around 737 nm, as displayed in Fig. 1a (transitions labelled from A to D). This spectral signature originates from the doubly split ground and excited states shown in Fig. 1b [33] , [34] . An applied magnetic field further lifts any degeneracies of these four transitions, as can be seen in Fig. 1c for a single SiV − centre in a nanocrystal (blue spectrum), and for an ensemble of SiV − centres in bulk diamond (red spectrum). Common to both spectra is the measured quadruplet splitting in the optical transitions, which is consistent with an energy level scheme based on spin-1/2 ground and excited states ( Fig. 1d ) [35] . Theoretical analysis based on density functional theory [28] , as confirmed by a recent ab initio study [36] , has determined a D 3d symmetry for the SiV − centre and assigned the optical ground and excited states to E g and E u states, respectively. The system can then be described by a Hamiltonian comprising orbital and spin Zeeman terms, the Jahn–Teller effect, which partially lifts the orbital degeneracies and a spin-orbit coupling term ( L·S ). Group theoretic analysis predicts that, in the case of the SiV − centre, only the L z S z component (z along the C 3 axis of the centre, that is, the [111] axis of the lattice) of the spin-orbit operator acts on the E g and E u states [31] , providing an inherent quantization axis along the 111 directions but leaving the spin as a good quantum number analogous to the NV − centres [37] . The degree of spin mixing introduced by the Jahn–Teller and Zeeman parts of the Hamiltonian can be quantified by defining spin purity as the probability of finding a state in one given spin projection m s =±1/2 only. Resonance fluorescence at 0 T Resonance fluorescence through state-selective excitation is a powerful tool to reveal the internal structure of quantum emitters. 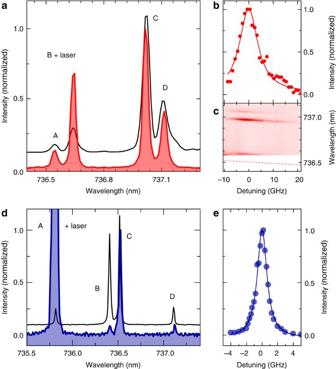Figure 2: Resonance fluorescence at 0 T. (a) Resonance fluorescence spectrum at 4 K for a SiV−ensemble (red shaded curve) with laser resonantly driving transition B, and non-resonant spectrum (black solid curve). (b) Photoluminescence excitation of transition A for a SiV−ensemble. The maximum intensity of transition C is plotted as a function of the resonant laser detuning (red dots) and can be fitted by a single Lorentzian (red solid curve) with full width at half maximum (FWHM) 9.1±0.7 GHz. (c) As the laser is tuned towards lower wavelengths across transition A (red dashed line), the observed fluorescing transition wavelengths B–C exhibit the same blue shift in the spectrum. Consequently, for a given laser frequency only a subensemble of the centres with identical strain conditions is excited. (d) Resonance fluorescence spectrum at 4 K for a single SiV−in nanodiamond (confirmed via photon correlation measurements), with laser resonantly exciting transition A (blue shaded curve) and non-resonant spectrum (black solid curve). The relative intensities of transitions under resonant excitation differ from the ones obtained in the non-resonant spectrum owing to the polarization-based laser suppression (seeSupplementary Fig. 5). (e) Photoluminescence excitation of transition A for the same single centre in nanodiamond. The maximum intensity of peak C is plotted as a function of laser detuning (blue dots) and can be fitted by a single Lorentzian (blue solid curve) with FWHM of 1.4±0.1 GHz. We first study an ensemble of SiV − centres in a low-strain bulk diamond at 0 T. Figure 2a displays the SiV − spectrum (red curve) observed when driving transition B resonantly (as labelled in Fig. 1a ). Here the laser is suppressed by polarization rejection (see Methods) and contributes only a small fraction to the full spectrum (see Methods and Supplementary Fig. 1 ). Although resonant excitation selectively populates one excited state branch, all four transitions are visible indicating a relaxation process between the excited state branches before photon emission. Tuning the laser frequency across transition A, while monitoring the fluorescence of transition C in the spirit of photoluminescence excitation, reveals the absorption profile of transition A (solid red circles in Fig. 2b ). The extracted full width at half maximum of ~10 GHz is consistent with the inhomogenous broadening of the ensemble under non-resonant excitation [32] due to residual strain in the sample (as evidenced by the shift of transitions along with laser frequency in Fig. 2c ). For a single centre in a nanodiamond, the fluorescence spectrum, obtained by driving transition A resonantly, is shown in Fig. 2d (blue curve). Owing to the strain in the crystal, the transitions of this centre are shifted beyond the inhomogenous broadening of the ensemble in bulk diamond, such that the exact spectrum varies from centre to centre. The absorption linewidth of 1.4 GHz for this transition ( Fig. 2e ) is only an order of magnitude above the radiatively broadened limit (~100 MHz) [22] , [33] , which should be reachable straightforwardly using impurity-free diamond substrates, as was shown for NV centres [38] . This linewidth also marks the minimum Zeeman splitting needed to resolve spin sublevels spectrally under resonant excitation. Figure 2: Resonance fluorescence at 0 T. ( a ) Resonance fluorescence spectrum at 4 K for a SiV − ensemble (red shaded curve) with laser resonantly driving transition B, and non-resonant spectrum (black solid curve). ( b ) Photoluminescence excitation of transition A for a SiV − ensemble. The maximum intensity of transition C is plotted as a function of the resonant laser detuning (red dots) and can be fitted by a single Lorentzian (red solid curve) with full width at half maximum (FWHM) 9.1±0.7 GHz. ( c ) As the laser is tuned towards lower wavelengths across transition A (red dashed line), the observed fluorescing transition wavelengths B–C exhibit the same blue shift in the spectrum. Consequently, for a given laser frequency only a subensemble of the centres with identical strain conditions is excited. ( d ) Resonance fluorescence spectrum at 4 K for a single SiV − in nanodiamond (confirmed via photon correlation measurements), with laser resonantly exciting transition A (blue shaded curve) and non-resonant spectrum (black solid curve). The relative intensities of transitions under resonant excitation differ from the ones obtained in the non-resonant spectrum owing to the polarization-based laser suppression (see Supplementary Fig. 5 ). ( e ) Photoluminescence excitation of transition A for the same single centre in nanodiamond. The maximum intensity of peak C is plotted as a function of laser detuning (blue dots) and can be fitted by a single Lorentzian (blue solid curve) with FWHM of 1.4±0.1 GHz. Full size image Spin-tagged fluorescence of unstrained SiV − centres Applying a magnetic field of 4 T to the ensemble of SiV − centres in bulk diamond allows us to address excited states with a given spin orientation selectively. First, we drive the transition labelled A2 (see Supplementary Fig. 2 ) to populate a Zeeman sublevel of the upper branch of the excited state, expected theoretically to be a spin-up projection, as shown in Fig. 3a (ref. 31 ). The resulting spectrum, shown in Fig. 3b (red shaded curve), is strikingly different from the spectrum obtained under non-resonant excitation ( Fig. 3c ); only half of the available optical transitions are visible and they originate from two excited states only. This is in stark contrast to thermal distribution at 4 K, which would lead to a finite population probability for all excited states. Here the relaxation process in the excited state takes place only between the two sublevels with the same Zeeman response, that is, same spin projection. To populate an excited state sublevel with the opposite Zeeman response, expected theoretically to be a spin-down projection, we resonantly drive transition B3 (blue double arrow in Fig. 3d ). The resulting spectrum, shown in Fig. 3e (blue shaded curve), is strongly anti-correlated with that in Fig. 3b , and the sum of the two spectra produces the full spectrum observed under non-resonant excitation ( Fig. 3c ). The spectra in Fig. 3b,e further reveal that from the populated excited states, optical transitions to all ground states occur, irrespective of their spin projection. The anti-correlation in the spectra arises from the high degree of spin purity in the excited state, that is, a high probability of finding each excited state in one of the two spin states only. In contrast, what appears as a violation of spin preservation in the optical transitions is a consequence of the orientation of the applied magnetic field affecting mostly the electronic ground state. Indeed, when the magnetic field is not parallel to the SiV − axis (as is the case in our experiment, see Methods) the original quantization axis of the centre is tilted because of the magnetic field-induced non-diagonal terms in the spin-orbit basis, which in turn induces an apparent spin mixing. With an angle of 54.7° between the 111 SiV − axes and the 4-T magnetic field along [001] (see Supplementary Fig. 3 ), the spin-orbit coupling strength in the excited state is still dominant and the spin-projection sublevel in the higher-lying excited state sustains a spin purity of 97% (Hepp et al. [31] ), which agrees well with the 4.1±1.2% overlap between the two anti-correlated spectra of Fig. 3 (see Methods and Supplementary Fig. 4 ). On the other hand, the spin-orbit coupling strength in the ground state is comparable to the off-axis contributions of the Zeeman Hamiltonian (at 4 T) resulting in a degree of spin purity ranging from 50 to 80% for the ground-state branches [31] . This effective spin mixing gives rise to finite intensity in all optical transitions starting from a given excited state. 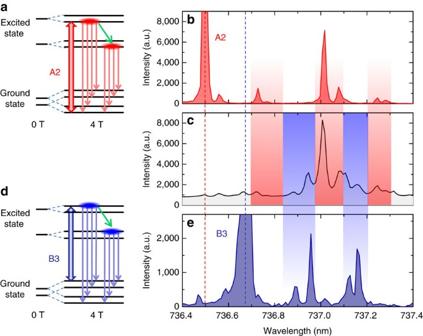Figure 3: Resonance fluorescence of ensemble SiV−at 4 T. (a) Energy level scheme for a SiV−in bulk diamond at 0 and 4 T. The driven transition populates the spin-down projection in the upper branch of the excited states and is indicated by a red double arrow. Relaxation takes place to the spin-down projection in the lower branch of the excited states as indicated by the green arrow. The thin red arrows indicate the transitions observed in the spectrum in panelb. (b) Resonance fluorescence spectrum measured driving transition A2 at 4 T for an SiV−ensemble in bulk diamond (red shaded curve). (c) Non-resonant fluorescence spectrum at 4 T for an SiV−ensemble (black solid curve). (d) Energy level scheme for a SiV−in bulk diamond at 0 and 4 T. The driven transition populates the spin-up projection in the upper branch of the excited state and is indicated by a blue double arrow. Relaxation takes place to the spin-up projection in the lower branch of the excited state as indicated by the green arrow. The thin blue arrows indicate the transitions observed in the resonant spectrum (e). (e) Resonance fluorescence spectrum measured when driving transition B3 at 4 T for an SiV−ensemble (blue shaded curve). The fluorescing transitions inbandeare highlighted with red and blue panels, respectively, on the non-resonant spectrum inc. The laser wavelengths used for resonant excitation inbandeare indicated with red and blue dashed lines, respectively. Figure 3: Resonance fluorescence of ensemble SiV − at 4 T. ( a ) Energy level scheme for a SiV − in bulk diamond at 0 and 4 T. The driven transition populates the spin-down projection in the upper branch of the excited states and is indicated by a red double arrow. Relaxation takes place to the spin-down projection in the lower branch of the excited states as indicated by the green arrow. The thin red arrows indicate the transitions observed in the spectrum in panel b . ( b ) Resonance fluorescence spectrum measured driving transition A2 at 4 T for an SiV − ensemble in bulk diamond (red shaded curve). ( c ) Non-resonant fluorescence spectrum at 4 T for an SiV − ensemble (black solid curve). ( d ) Energy level scheme for a SiV − in bulk diamond at 0 and 4 T. The driven transition populates the spin-up projection in the upper branch of the excited state and is indicated by a blue double arrow. Relaxation takes place to the spin-up projection in the lower branch of the excited state as indicated by the green arrow. The thin blue arrows indicate the transitions observed in the resonant spectrum ( e ). ( e ) Resonance fluorescence spectrum measured when driving transition B3 at 4 T for an SiV − ensemble (blue shaded curve). The fluorescing transitions in b and e are highlighted with red and blue panels, respectively, on the non-resonant spectrum in c . The laser wavelengths used for resonant excitation in b and e are indicated with red and blue dashed lines, respectively. Full size image Spin-tagged fluorescence of strained single SiV − centres We now investigate the influence of strain through resonance fluorescence from a single centre located in a nanodiamond. A magnetic field of 2 T allows us to optically resolve the individual transitions of the centre shown in Fig. 1c . The excitation laser is brought into resonance with transition A1 (as shown in Fig. 4a ) and transition A2. This leads to fluorescence spectra with selective population of the spin-up (blue curve) and spin-down (red curve) sublevels in the higher branch of the excited state, respectively, as seen in Fig. 4b . The signature of spin selectivity demonstrated in bulk is only partially observed in the resulting fluorescence spectra shown in Fig. 4b . While the transitions B1–B4, originating directly from the higher-lying branch of the excited state, still exhibit a high degree of spin selectivity (hence spin purity), the transitions C1–D4, which originate from the lower branch after a relaxation step, do not display such spin selectivity. This breakdown is induced by the strong strain field not oriented with the symmetry axis of the centre. This can be understood based on the model presented in (Hepp et al. [31] ), where an additional term for the strain perturbation is added to the total Hamiltonian to account for the strain field in the nanodiamonds (not discussed here). 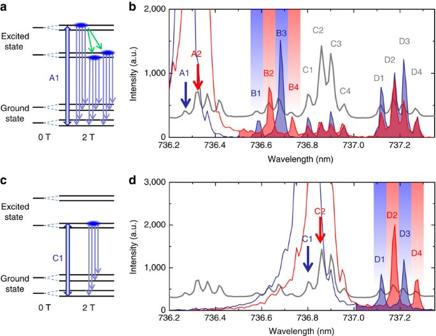Figure 4: Resonance fluorescence at 2 T for a single SiV−in nanodiamond. (a) Energy level scheme for the single SiV−in nanodiamond at 0 and 2 T. Driving transition A1 (indicated by a blue double arrow) results in populating the spin-up sublevel in the upper branch of the excited state. From there, relaxation takes place to both lower branch sublevels (green arrows). The spectrum obtained when driving this transition is shown in panelb(blue shaded curve), along with a spectrum when resonantly driving transition A2, which populates the spin-down projection sublevel (red shaded curve). Driven transitions are indicated in the spectra by the red and blue arrows on the non-resonant spectrum (grey curve). (c) Same as panela, but when driving transition C1 (blue double arrow), populating the spin-up sublevel in the lower branch. (d) The spectra obtained when driving C1 (blue shaded curve) and C2 (red shaded curve) along with the spectrum obtained under non-resonant excitation (grey curve). Figure 4: Resonance fluorescence at 2 T for a single SiV − in nanodiamond. ( a ) Energy level scheme for the single SiV − in nanodiamond at 0 and 2 T. Driving transition A1 (indicated by a blue double arrow) results in populating the spin-up sublevel in the upper branch of the excited state. From there, relaxation takes place to both lower branch sublevels (green arrows). The spectrum obtained when driving this transition is shown in panel b (blue shaded curve), along with a spectrum when resonantly driving transition A2, which populates the spin-down projection sublevel (red shaded curve). Driven transitions are indicated in the spectra by the red and blue arrows on the non-resonant spectrum (grey curve). ( c ) Same as panel a , but when driving transition C1 (blue double arrow), populating the spin-up sublevel in the lower branch. ( d ) The spectra obtained when driving C1 (blue shaded curve) and C2 (red shaded curve) along with the spectrum obtained under non-resonant excitation (grey curve). Full size image Bypassing the interbranch relaxation mechanism by directly populating a spin sublevel of the lower branch allows us to access the degree of spin purity in this branch. This is illustrated in Fig. 4c for the case of populating the spin-up sublevel. Phonon-assisted excitation to the upper branch is strongly suppressed at 4 K owing to the large energy difference between the two branches for this centre. In the resulting spectra, shown in Fig. 4d , the transitions resonantly populating spin-up and spin-down sublevels are indicated by blue and red arrows, respectively. Under these conditions, the contrast between fluorescence intensity originating from the two spin orientations (red and blue filled curves) is recovered to above 90%. This evidences high-spin purity within both excited state branches. Therefore, by selecting the driven transitions, spin-selective optical access to SiV − centres can be achieved in strained nanodiamonds as well as low-strain bulk diamond. A natural extension of this work is to align the C 3 symmetry axis of a SiV − centre to the magnetic field either by rotating the samples (which was technically not possible in our set-up) or by implanting SiV − centres in a [111]-oriented diamond crystal. Both approaches are expected to restore more than 90% spin purity in the ground state and near-unity spin purity in the excited state eliciting the inherent optical selection rules linked to the spin orientation. These properties mark the SiV − centre desirable for all applications that require optical access to well-defined spin states. All-optical ultrafast spin manipulation techniques or optically detected magnetic resonance can then give access to the electronic spin coherence of the pure ground state. Full coherent control of the SiV − spin state along with fluorescence-detection-based spin initialization and read-out will be within reach for the realization of a highly efficient spin-photon quantum interface. Sample fabrication The ensemble of SiV − centres in bulk was grown using a hot filament chemical vapour deposition technique [33] , where SiV − centres are created in situ owing to residual silicon contamination of the CVD reactor. A Ib high pressure high temperature diamond (Sumitomo) with [001] orientation was used as a substrate, and was overgrown with a high-quality diamond film. The homoepitaxial growth minimizes stress arising from thermal expansion mismatch of substrate and diamond, and helps reduce dislocations in the grown diamond lattice. High crystalline quality is achieved by applying optimized growth conditions involving a low methane fraction (0.26% CH 4 in H 2 ) and slow growth. The thickness of the diamond film of 80–100 nm was estimated by growing a diamond film on a non-diamond substrate with identical growth conditions where the thickness could easily be measured. Single SiV − centres in nanodiamonds were CVD grown on a silicon substrate, which was covered by an intermediate yttria-stabilized-zirconia buffer layer and atop a 150-nm iridium layer [14] . This iridium layer allows for optimized growth conditions, and reduces the amount of silicon incorporated into the nanodiamonds from the substrate during growth. Before growth, the substrate is seeded with deagglomerated synthetic nanodiamonds with sizes up to 30 nm (Microdiamant Liquid Diamond MSY). The aqueous solution of these diamonds is diluted appropriately to achieve a seed density of roughly 2.5 seeds per μm 2 . The density of crystals containing SiV − centres is estimated to be around one per 50 × 50 μm 2 . The seeded substrates were exposed to microwave plasma-assisted CVD process for 25 min, using a hydrogen-plasma containing 1% methane. The gas pressure was 30 mbar and the microwave power was 2,000 W. These conditions resulted in a crystal size of about 130 nm with a s.d. of 30 nm. Confocal microscope set-up The sample is mounted on a piezo-driven three-axis translation stage (attocube ANPz 101/LT and two ANPx 101/LT) in a helium bath cryostat ( T =4.2 K) at the centre of a fixed orientation, tunable 7 T superconducting magnet (Cryogenic) in Faraday configuration. Excitation of the SiV − centres is performed non-resonantly at 700 nm (Coherent Mira 900-CW) and resonantly using a frequency-tunable external-cavity diode laser around 737 nm (Toptica DL 100 Pro Design). SiV − spectra were recorded using a spectrometer with ~40 μeV resolution (PI Acton). All measurements are performed using a fibre-based confocal microscope with polarization-controlled excitation and collection (polarizers: Thorlabs LPVIS050-MP, half-wave plates: Thorlabs AHWP05M-980). Light is focused onto the sample with a numerical aperture=0.68 aspheric lens (Thorlabs C330TME-B), and residual laser light in the detection arm is removed with either a 720-nm longpass filter (third millennium) or with a polarizer set perpendicularly to the incoming laser polarization. With the latter technique, laser suppression up to 5 × 10 −7 was reached. Determination of the photon ratio In the resonant spectrum of Fig. 2a , the integrated intensity of each transition is evaluated through Lorentzian fits (see Supplementary Fig. 1a with the following results: I (A)=0.14, I (B)+ I (laser)=0.66, I (C)=1.0, I (D)=0.46 (the intensities are normalized to that of transition C. Uncertainties on fits are below 0.01 for all transitions). First, a lower bound can be set by assuming that no emission from transition B is collected ( I (B)=0). With this assumption, a ratio between laser and SiV − emission of 1:2.4 is obtained. Next, we evaluate I (B) when this transition is driven. The intensities in the resonant spectrum can be compared with the respective ones for non-resonant excitation ( Fig. 1a ), labelled as I ′. These are I′ (A)=0.058, I′ (B)=0.20, I′ (C)=1.0 and I′ (D)=0.46. The ratios I/I′ differ for transitions A, C and D, with values ranging from 0.43 to 1.00. Assuming that I (B)/ I′ (B) lies within that range, the intensity of transition B in the resonant case can be expected between 0.20 and 0.47. This leads to an intensity ratio of the laser to SiV − emission between the extrema of 1:3.9 and 1:11. Another way of evaluating the intensity of transition B when resonantly driven is by applying the same method of intensity comparison with the spectrum where transition A is resonantly excited, knowing that transitions A and B share the same excited state. In the spectrum with A driven resonantly (see Supplementary Fig. 1b ), the following intensities I″ are obtained: I″ (B)=0.33, I″ (C)=1 and I″ (D)=0.27. The ratios I/I″ range from 0.59 to 1.00, resulting in the intensity of transition B being between 0.33 and 0.57. This finally leads to a ratio between laser and SiV − emission ranging from 1:5.9 to 1:24. Contrast between transition subsets under excitation Here we describe how we can extract information about the degree of spin conservation in the excited state by comparing transition intensities when populating spin-up and spin-down excited states by driving transitions A2 and B3, respectively ( Fig. 3b,e ). For this analysis, we restrict ourselves to intensities in transitions C1 to D4, originating from the lower-lying excited state. This is to exclude contributions from the excitation laser. Visual inspection of the spectra in Supplementary Fig. 4 (red curve for driving transition A2 and blue curve when driving transition B3) shows that when populating the spin-down excited states (red spectrum), contributions to transitions originating from spin-up excited states are within the noise of the spectrum. In contrast, when populating the spin-up excited states (blue spectrum), a finite contribution into the ‘forbidden’ transition C2 is visible. We use this intensity to estimate the branching ratio of the relaxation mechanism in the excited state. We now consider the blue spectrum in Supplementary Fig. 4 . According to Fermi’s golden rule, the transition rate Г for a specific transition is given by , where ħ is the reduced Planck’s constant, ρ i is the probability of finding the system in the excited state at the origin of the transition, ϕ i is the electronic wavefunction of the excited state, D is the dipole operator and ϕ f is the electronic wavefunction in the ground state. If we assume that the dipole matrix element is constant for all transitions, then the transition rates become proportional to the populations ρ i in the excited state and give access to the branching ratios between the two spin states. This assumption is not entirely correct, but since C2 is the brightest transition under non-resonant excitation, the transition matrix element will be larger. Consequently, the branching ratio will be overestimated when considering the blue spectrum yielding a lower limit for spin conservation. Focusing on the blue spectrum for the spin-down transitions, the transitions can be fitted with a series of five Lorentzians (blue shaded curve in Supplementary Fig. 4 ): four for the ‘allowed’ transitions C1, D1, C3 and D3, and one for the ‘forbidden’ transition C2. The other ‘forbidden’ transitions are too weak to be considered. The intensity ratio between transition C2 and the total emission into the five transitions is 3±1.2%. The additional error made by neglecting the intensities into the forbidden transitions D2, C4 and D4 can be calculated by considering the respective intensities in the red spectrum. A Lorentzian fit of the four visible transitions reveals that transition C2 constitutes 73.2±0.9% of the total red spectrum. Therefore, the branching ratio between transitions C2, D2, C4 and D4 (the forbidden ones) and transitions C1, D1, C3 and D3 is 4.1±1.2%, confirming the strong spin conservation of the relaxation mechanism in the excited state for centres in bulk diamond. How to cite this article: Müller, T. et al. Optical signatures of silicon-vacancy spins in diamond. Nat. Commun. 5:3328 doi: 10.1038/ncomms4328 (2014).